Akt-p53-miR-365-cyclin D1/cdc25A axis contributes to gastric tumorigenesis induced by PTEN deficiency Although PTEN/Akt signaling is frequently deregulated in human gastric cancers, the in vivo causal link between its dysregulation and gastric tumorigenesis has not been established. Here we show that inactivation of PTEN in mouse gastric epithelium initiates spontaneous carcinogenesis with complete penetrance by 2 months of age. Mechanistically, activation of Akt suppresses the abundance of p53, leading to decreased transcription of miR-365, thus causing upregulation of cyclin D1 and cdc25A, which promotes gastric cell proliferation. Importantly, genetic ablation of Akt1 restores miR-365 expression and effectively rescues gastric tumorigenesis in PTEN -mutant mice. Moreover, orthotopic restoration of miR-365 represses PTEN -deficient-induced hyperplasia. In human gastric cancer tissues, miR-365 reduction correlates with poorly differentiated histology, deep invasion and advanced stage, as well as the deregulation of PTEN, phosphorylated Akt, p53, cyclin D1 and cdc25A. These data demonstrate that the PTEN-Akt-p53-miR-365-cyclin D1/cdc25A axis serves as a new mechanism underlying gastric tumorigenesis, providing potential new therapeutic targets. Gastric cancer (GC) is the fourth most frequently occurring malignancy, exhibiting considerable geographic variation and ranks as the second leading cause of cancer-related deaths [1] . GC results from a combination of environmental factors and the accumulation of generalized and specific genetic alterations [2] . Although accumulating evidence shows that various genetic alterations cause tumorigenesis and progression of GC [3] , the molecular mechanisms underlying the pathogenesis of gastric carcinomas remain to be fully defined. Phosphatase and tensin homologue deleted on chromosome 10 (PTEN) is a tumour suppressor that regulates cell survival and proliferation by antagonizing phosphatidylinositol 3-kinase/protein kinase B (PKB/Akt) signaling [4] . In human GC, loss of heterozygosity of PTEN [5] , [6] , reduced expression of PTEN [7] , [8] , [9] and overexpression of phosphorylated Akt (p-Akt) [10] , [11] , [12] are frequently correlated with tumour progression and poor prognosis. In vitro studies have shown that activation of Akt signaling is responsible for gastric cell proliferation, invasiveness and metastasis [12] , [13] , [14] , [15] . However, the function of the PTEN/Akt pathway during gastric tumorigenesis is poorly investigated. MicroRNAs (miRNAs) are small, non-coding, single-stranded RNAs that suppress gene expression post-transcriptionally primarily through sequence-specific interaction with the 3′-untranslated regions (UTRs) of cognate mRNA targets [16] . miRNAs have been associated with a wide range of physiological and pathological processes, including tumour formation and progression [17] . miRNAs are frequently deregulated in cancers, in which they function as a group to mark differentiation states or individually as bona fide oncogenes or tumour suppressors [18] . In the context of GC, recent reports show that characteristic miRNA signatures are closely associated with disease progression and clinical outcome [19] , [20] , [21] . Moreover, some miRNAs altered in GC have been verified to control GC cell proliferation, apoptosis and inflammation [22] , [23] . However, the mechanism underlying the deregulation of miRNA expression in GC remains unclear. Recent studies have revealed that miRNAs could mediate the oncogenic function of the Akt pathway in several cellular processes, including cell proliferation, epithelial–mesenchymal transition and tumour angiogenesis, in breast, colon and lung cancers [24] , [25] . It has been shown that the activation of Akt phosphorylates C/EBP-β or downregulates p53 abundance, both of which act as transcription factors to directly control miR-145 transcription [26] , [27] . However, the function of Akt-regulated miRNAs in gastric tumorigenesis has not been reported. Here we show that gastric epithelium-specific PTEN deficiency initiates gastric tumorigenesis in mice and demonstrate that deregulated PTEN-Akt-p53-miR-365-cyclin D1/cdc25A axis contributes to gastric tumorigenesis. PTEN deletion causes gastric tumorigenesis in mice To clarify whether PTEN is involved in gastric tumorigenesis, mice carrying floxed PTEN alleles [28] were bred with SP-A-Cre transgenic mice that express the Cre recombinase in gastric epithelium [29] to generate SP-A-Cre;PTEN flox/+ (control) and SP-A-Cre;PTEN flox/flox ( PTEN fl/fl ) mice. The efficiency and cell specificity of Cre-mediated recombination was confirmed by LacZ staining of gastric tissues from SP-A-Cre;ROSA26 double transgenic mice. Specific Cre-mediated recombination was detected in glandular epithelial cells of mouse stomach at embryonic day 18.5 ( Fig. 1a ). Cre-mediated excision of exons 4–5 of the PTEN gene in the gastric epithelium was confirmed using Southern blot analysis ( Supplementary Fig. S1a ). Western blot and immunohistochemical analyses showed that PTEN expression was observed in the gastric epithelium from control mice but was dramatically decreased in the SP-A-Cre;PTEN fl/fl epithelium ( Fig. 1b ; Supplementary Fig. S1b ). Conversely, p-Akt expression was undetectable in control epithelium but was dramatically elevated in PTEN -deficient epithelium ( Fig. 1b ; Supplementary Fig. S1b ). The data indicated that PTEN was efficiently disrupted, and consequently Akt activation was triggered in gastric epithelium. 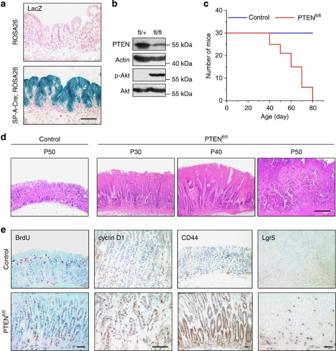Figure 1: Disruption ofPTENin mouse gastric epithelium results in tumorigenesis. (a) LacZ staining ofROSA26 and SP-A-Cre;ROSA26glandular epithelium at embryonic day 18.5. (b) Western blot analysis of the expressions of PTEN and p-Akt inPTEN-mutant and control gastric epithelium at P20 (n=4). (c) Survival curves ofPTEN-mutant (red) and control (blue) mice (n=30). (d) Hematoxylin and eosin staining (HE) of gastric epithelium from 50-day-old control along with 30-day-, 40-day- and 50-day-oldPTEN-mutant mice (n=5–10). (e) Immunohistochemical analysis of BrdU, cyclin D1 and CD44, andin situhybridization analysis of Lgr5 in 40-day-oldSP-A-Cre;PTENfl/fl(PTENfl/fl) andSP-A-Cre;PTENfl/+(Control) gastric epithelium (n=5–10). Scale bars represent 25 μm in (a) and (e), 100 μm in (d). Figure 1: Disruption of PTEN in mouse gastric epithelium results in tumorigenesis. ( a ) LacZ staining of ROSA26 and SP-A-Cre;ROSA26 glandular epithelium at embryonic day 18.5. ( b ) Western blot analysis of the expressions of PTEN and p-Akt in PTEN -mutant and control gastric epithelium at P20 ( n= 4). ( c ) Survival curves of PTEN- mutant (red) and control (blue) mice ( n= 30). ( d ) Hematoxylin and eosin staining (HE) of gastric epithelium from 50-day-old control along with 30-day-, 40-day- and 50-day-old PTEN -mutant mice ( n= 5–10). ( e ) Immunohistochemical analysis of BrdU, cyclin D1 and CD44, and in situ hybridization analysis of Lgr5 in 40-day-old SP-A-Cre;PTEN fl/fl ( PTEN fl/fl ) and SP-A-Cre;PTEN fl/+ (Control) gastric epithelium ( n= 5–10). Scale bars represent 25 μm in ( a ) and ( e ), 100 μm in ( d ). Full size image All SP-A-Cre;PTEN fl/fl mice exhibited progressive weakness and loss of body weight after the age of 1 month. The anatomy of SP-A-Cre;PTEN fl/fl mice at P50 (50 postnatal days) revealed that their stomachs were markedly enlarged and thickened compared with control mice ( Supplementary Fig. S1c ). SP-A-Cre;PTEN fl/fl mice died between P40 and P80 ( Fig. 1c ) possibly due to gastric outlet obstruction and consequent malnutrition. Histological examination of glandular epithelium from control mice at P50 revealed very clearly defined gastric units ( Fig. 1d ). In contrast, PTEN -mutant mice presented markedly hyperplastic epithelium as early as P30, which was characteristic of elongated gastric units with single-layered cells ( Fig. 1d ). By P40, gastric dysplasia characterized by multiple-layered cells in gastric units with the loss of cellular polarity was evident in all mutant mice ( Fig. 1d ). Thereafter, intramucosal or early gastric carcinoma, which represented severe dysplasia involving the entire thickness of gastric epithelium and abnormal glandular structures resulting from branching and interglandular bridging, was progressively present in PTEN -mutant mice ( Fig. 1d ). In particular, we found a small proportion of PTEN -mutant mice (2/30) that displayed well-differentiated, invasive adenocarcinoma in the submucosa, which was further confirmed with Alcian blue staining ( Supplementary Fig. S1d ). We also analysed the histology of the brain, lung and intestine from 60-day-old SP-A-Cre;Pten fl/fl mice, in which PTEN was also deleted driven by SP-A-Cre ( Supplementary Fig. S1e ), and found no obvious abnormality in these tissues ( Supplementary Fig. S1f ). We next investigated whether the marked hyperplasia in PTEN -mutant epithelium was due to enhanced cellular proliferation. BrdU-labelling results showed that replicating cells in the normal epithelium were localized in the neck zone, where the gastric progenitors resided ( Fig. 1e ). In PTEN -mutant mice at P40, BrdU-positive cells were significantly increased in an extensive pattern throughout the mucosa ( Fig. 1e ). We found that the nuclear expression of cyclin D1, a well-known downstream effector of the Akt pathway, was significantly increased in the PTEN -mutant epithelium ( Fig. 1e ). Furthermore, we found that the expression of CD44 and Lgr5, two identified markers for gastric stem-like cells [30] and stem cells [31] , respectively, was obvious in PTEN -deficient corpus epithelium but undetectable in the control epithelium at P40 ( Fig. 1e ). We further tested whether abnormal epithelial proliferation was accompanied by differentiation defects in PTEN mutants. To distinguish the main epithelial cell types in gastric units, the expression levels of differentiation markers ulex europaeus agglutinin (UEA) for pit cells, dolichos biflorus agglutinin (DBA) for parietal cells, griffonia simplicifolia II for mucous neck cells and pepsinogen II for chief cells were examined. At P40, the terminally differentiated cells, except for some pit cells, were almost undetectable in PTEN mutants ( Supplementary Fig. S1g ). These results demonstrated that PTEN deficiency increased cell proliferation, blocked terminal differentiation and eventually led to tumorigenesis in the gastric epithelium. miR-365 inhibits gastric cancer cell proliferation To explore the role of miRNAs in gastric tumour formation caused by PTEN deletion, we compared miRNA expression profiles between PTEN- deficient and control epithelia ( Fig. 2a ). The expression of the deregulated miRNAs was confirmed using northern blot or real-time quantitative PCR (qRT–PCR) ( Fig. 2b ; Supplementary Fig. S2a,b ). 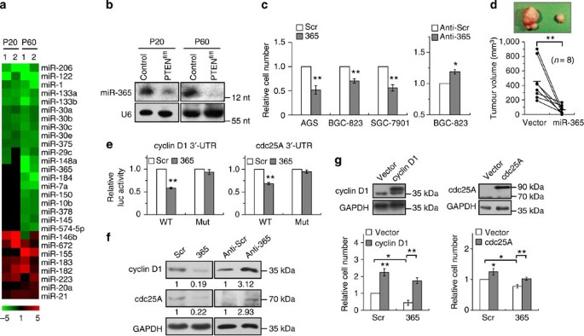Figure 2: miR-365 suppresses gastric cancer cell proliferation by targeting cyclin D1 and cdc25A. (a) Profiling data of the upregulated (red) and downregulated (green) miRNAs inPTEN-mutant gastric epithelium at P20 and P60 (mean change fold >2;P<0.01, Student’st-test). (b) The expression of miR-365 inPTEN-mutant and control epithelium at P20 and P60 was measured using northern blot analysis (n=4). (c) Cell viability was determined by cell count. Gastric cancer cell lines AGS, BGC-823 and SGC-7901 were transfected with miR-365 (365) or scrambled (Scr) mimic for 72 h (n=4–8). BGC-823 cells were transfected with miR-365 antisense oligonucleotides (anti-365) or scrambled antisense oligonucleotides (anti-Scr) for 72 h (n=4). (d) Tumour formation assay of stably miR-365-expressing (miR-365) and control (vector) BGC-823 cells in a mouse xenograft (n=8). Photographs illustrated representative feature of tumour growth ~4 weeks after injection. Tumour growth was determined by tumour volume. The lines between controls and miR-365-overexpressing xenograft tumours represented the connected data from the corresponding sides of the same nude mouse. **P<0.01 was calculated using Pair-Samplet-test. (e) Luciferase reporter activities of reporter constructs. BGC-823 cells were cotransfected with the reporter constructs containing wild-type (WT) 3′-UTRs of cyclin D1 or cdc25A, as well as mutant (Mut) 3′-UTRs with the putative target sites mutated (As illustrated inSupplementary Fig. S2p), together with miR-365 or scrambled mimic (n=6). (f) The protein levels of cyclin D1 and cdc25A were determined using western blot analysis. BGC-823 cells were transfected with miR-365 (365) or scrambled (Scr) mimic as well as miR-365 (anti-365) and scrambled (anti-Scr) antisense oligonucleotides (n=6). (g) Cell viability was determined by cell count. BGC-823 cells were cotransfected with miR-365 mimic and pCMV-HA-cyclin D1 or pCMV6-cdc25A-GFP construct for 24 h (n=3). The upper bands in western blot indicated the exogenous expression of cyclin D1 or cdc25A. The lower bands indicated the endogenous ones. Values represent the mean±s.d. *P<0.05 and **P<0.01 were calculated using Student’st-test. Figure 2: miR-365 suppresses gastric cancer cell proliferation by targeting cyclin D1 and cdc25A. ( a ) Profiling data of the upregulated (red) and downregulated (green) miRNAs in PTEN -mutant gastric epithelium at P20 and P60 (mean change fold >2; P <0.01, Student’s t -test). ( b ) The expression of miR-365 in PTEN -mutant and control epithelium at P20 and P60 was measured using northern blot analysis ( n= 4). ( c ) Cell viability was determined by cell count. Gastric cancer cell lines AGS, BGC-823 and SGC-7901 were transfected with miR-365 (365) or scrambled (Scr) mimic for 72 h ( n= 4–8). BGC-823 cells were transfected with miR-365 antisense oligonucleotides (anti-365) or scrambled antisense oligonucleotides (anti-Scr) for 72 h ( n= 4). ( d ) Tumour formation assay of stably miR-365-expressing (miR-365) and control (vector) BGC-823 cells in a mouse xenograft ( n= 8). Photographs illustrated representative feature of tumour growth ~4 weeks after injection. Tumour growth was determined by tumour volume. The lines between controls and miR-365-overexpressing xenograft tumours represented the connected data from the corresponding sides of the same nude mouse. ** P <0.01 was calculated using Pair-Sample t -test. ( e ) Luciferase reporter activities of reporter constructs. BGC-823 cells were cotransfected with the reporter constructs containing wild-type (WT) 3′-UTRs of cyclin D1 or cdc25A, as well as mutant (Mut) 3′-UTRs with the putative target sites mutated (As illustrated in Supplementary Fig. S2p ), together with miR-365 or scrambled mimic ( n= 6). ( f ) The protein levels of cyclin D1 and cdc25A were determined using western blot analysis. BGC-823 cells were transfected with miR-365 (365) or scrambled (Scr) mimic as well as miR-365 (anti-365) and scrambled (anti-Scr) antisense oligonucleotides ( n= 6). ( g ) Cell viability was determined by cell count. BGC-823 cells were cotransfected with miR-365 mimic and pCMV-HA-cyclin D1 or pCMV6-cdc25A-GFP construct for 24 h ( n= 3). The upper bands in western blot indicated the exogenous expression of cyclin D1 or cdc25A. The lower bands indicated the endogenous ones. Values represent the mean±s.d. * P <0.05 and ** P <0.01 were calculated using Student’s t -test. Full size image We filtered the candidate miRNAs whose expressions were deregulated in PTEN -mutant mice and changed upon treatment with the Akt pathway activator and inhibitors in GC cells ( Supplementary Fig. S2c–e ). miR-365 fulfilled these criteria. miR-365 was significantly downregulated in 20- and 60-day-old PTEN- mutant epithelia ( Fig. 2b ). Based on the role of PTEN in suppressing gastric tumorigenesis and the previously reported effect of miR-365 on cell proliferation in colon cancer cells [32] , we hypothesized that miR-365 could function as a tumour suppressor in GC. In human GC cell lines AGS, BGC-823 and SGC-7901, overexpression of miR-365 using a mimic ( Supplementary Fig. S2f,h ) significantly suppressed cell proliferation by 35–50% ( Fig. 2c ). Conversely, a 1.2-fold increase in cell numbers was observed in BGC-823 cells treated with miR-365 antisense oligonucleotides (anti-365) ( Fig. 2c ; Supplementary Fig. S2g,h ). Flow cytometric analysis revealed that miR-365 induced G1 arrest ( Supplementary Fig. S2i ) and had no effect on apoptosis ( Supplementary Fig. S2j ). Consistently, miR-365 overexpression dramatically reduced clonal growth by 50%, and knockdown of miR-365 increased clonal growth ( Supplementary Fig. S2k ). Additionally, stable overexpression of miR-365 in BGC-823 and AGS cells also decreased cell proliferation ( Supplementary Fig. S2l ), caused G1 arrest ( Supplementary Fig. S2m ), as well as inhibited clonal growth ( Supplementary Fig. S2n ). We further tested the potential of miR-365 for inhibiting gastric tumorigenesis. A soft agar colony formation assay revealed that stable overexpression of miR-365 in BGC-823 cells resulted in an ~80% reduction in colony numbers ( Supplementary Fig. S2o ), suggesting that miR-365 could inhibit cell proliferation in an anchorage-independent manner. Furthermore, miR-365 remarkably suppressed gastric tumorigenesis in a mouse xenograft model ( Fig. 2d ). We next dissected the potential mechanism underlying the inhibitory function of miR-365 in GC cell proliferation. Bioinformatics analysis using TargetScan revealed that the 3′-UTRs of cyclin D1 and cdc25A contain evolutionarily conserved miR-365-binding sites ( Supplementary Fig. S2p ). We focused on these two genes based on their roles in the transition through the G1/S checkpoint. The miR-365 mimic significantly inhibited the luciferase reporter activities of the wild-type 3′-UTR constructs of cyclin D1 and cdc25A in BGC-823 cells but not the mutant 3′-UTR constructs containing mutations in the complementary seed sites ( Fig. 2e ). In addition, miR-365 mimic markedly decreased the mRNA and protein levels of cyclin D1 and cdc25A ( Fig. 2f ; Supplementary Fig. S2q–s ). Conversely, knockdown of miR-365 clearly increased the concentration of cyclin D1 and cdc25A proteins ( Fig. 2f ). Furthermore, knockdown of cyclin D1 or cdc25A using short interfering RNA (siRNA) greatly repressed cell growth ( Supplementary Fig. S2t,u ). Overexpression of cyclin D1 or cdc25A rescued the miR-365-overexpressing phenotype of cell-growth inhibition ( Fig. 2g ), supporting the dominant role of these two factors in miR-365-mediated proliferation inhibition in GC cells. Taken together, these data demonstrated that miR-365 suppresses GC cell proliferation by inhibiting its targets cyclin D1 and cdc25A. miR-365 is negatively regulated by Akt signaling To further confirm that miR-365 was negatively regulated by Akt signaling, we assessed the change of miR-365 expression in response to Akt signaling stimuli. miR-365 expression was dramatically decreased upon treatment with fetal bovine serum (FBS), insulin or insulin-like growth factor 1 (IGF-1) in GC cell lines including BGC-823, AGS, NCI-N87 and PHM82 ( Fig. 3a ; Supplementary Fig. S3a–c ). Conversely, a dramatic increase in miR-365 expression was observed with the addition of phosphatidylinositol 3-kinase inhibitors LY294002 or Wortmannin ( Fig. 3b ; Supplementary Fig. S3d ). Furthermore, miR-365 was downregulated in BGC-823 and AGS cells transiently transfected with myristoylated Akt1 (Myr-Akt1), a constitutively active mutant of Akt1 ( Fig. 3c ; Supplementary Fig. S3e ). Conversely, miR-365 was upregulated by overexpression of kinase-deficient Akt1 (Akt1-KD) or by suppression of the endogenous Akt expression with siRNA ( Fig. 3c ; Supplementary Fig. S3e ). Finally, we utilized a luciferase reporter assay to assess whether the Akt pathway could regulate miR-365 transcription. The upstream 4-kb putative promoter of miR-193b-365 (refs 33 , 34 ) was cloned into a pGL4 basic vector to generate the reporter construct ( Supplementary Fig. S3f ). miR-193b-365 promoter activity was strikingly depressed upon activation of the Akt pathway by IGF-1 treatment or Myr-Akt1 overexpression and significantly enhanced by suppression of the Akt pathway with LY294002 addition or Akt1-KD transfection ( Fig. 3d ). The above data indicated that Akt signaling suppresses miR-365 transcription. 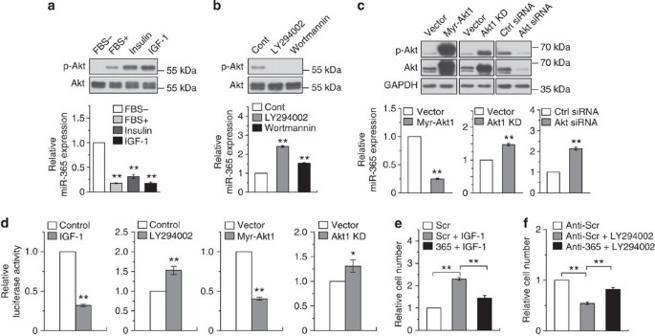Figure 3: miR-365 is inhibited by Akt signaling. (a–c) The relative level of miR-365 was measured using qRT–PCR. BGC-823 cells were treated with Akt pathway activators and inhibitors. Phosphorylation of Akt was verified using western blot analysis from the same cell lysates. (a) After 24-h starvation with 0.5% FBS (FBS−), cells were treated with 10% FBS (FBS+), 100 ng ml−1IGF-1 or 10 nM insulin for 24 h (n=4–6). (b) Cells were treated with 20 μM LY294002 or 100 nM Wortmannin for 12 h (n=4–6). (c) Cells were transfected with pUSE-Myr-Akt1 or pUSE-Akt1-KD plasmids as well as corresponding controls for 24 h or transfected with Akt1 siRNA as well as control siRNA for 48 h (n=4). (d) The luciferase reporter assay of miR-193b-365 promoter construct in BGC-823 cells after stimulation of IGF-1 or LY294002 as well as cotransfection with pUSE-Myr-Akt1 or pUSE-Akt1-KD plasmids (n=3–5). (e–f) Cell viability was determined by cell count in BGC-823 cells. (e) BGC-823 cells were pretreated with miR-365 (365) or scrambled (Scr) mimic for 24 h, followed by IGF-1 addition for another 48 h (n=5). (f) BGC-823 cells were pretreated with miR-365 (anti-365) or scrambled (anti-Scr) antisense oligonucleotides for 24 h, followed by LY294002 addition for another 24 h (n=4). Values represent the mean±s.d. *P<0.05 and **P<0.01 were calculated using Student’st-test. Figure 3: miR-365 is inhibited by Akt signaling. ( a – c ) The relative level of miR-365 was measured using qRT–PCR. BGC-823 cells were treated with Akt pathway activators and inhibitors. Phosphorylation of Akt was verified using western blot analysis from the same cell lysates. ( a ) After 24-h starvation with 0.5% FBS (FBS−), cells were treated with 10% FBS (FBS+), 100 ng ml −1 IGF-1 or 10 nM insulin for 24 h ( n= 4–6). ( b ) Cells were treated with 20 μM LY294002 or 100 nM Wortmannin for 12 h ( n= 4–6). ( c ) Cells were transfected with pUSE-Myr-Akt1 or pUSE-Akt1-KD plasmids as well as corresponding controls for 24 h or transfected with Akt1 siRNA as well as control siRNA for 48 h ( n= 4). ( d ) The luciferase reporter assay of miR-193b-365 promoter construct in BGC-823 cells after stimulation of IGF-1 or LY294002 as well as cotransfection with pUSE-Myr-Akt1 or pUSE-Akt1-KD plasmids ( n= 3–5). ( e – f ) Cell viability was determined by cell count in BGC-823 cells. ( e ) BGC-823 cells were pretreated with miR-365 (365) or scrambled (Scr) mimic for 24 h, followed by IGF-1 addition for another 48 h ( n= 5). ( f ) BGC-823 cells were pretreated with miR-365 (anti-365) or scrambled (anti-Scr) antisense oligonucleotides for 24 h, followed by LY294002 addition for another 24 h ( n= 4). Values represent the mean±s.d. * P <0.05 and ** P <0.01 were calculated using Student’s t -test. Full size image We next determined whether Akt signaling could promote cell proliferation by decreasing miR-365 expression. miR-365 mimic significantly abrogated the proliferative effect of the activated Akt pathway by treatment with IGF-1 or Myr-Akt1 ( Fig. 3e ; Supplementary Fig. S3g,h ). Conversely, knockdown of miR-365 attenuated the reduced cell growth caused by LY294002 ( Fig. 3f ). Consistently, fluorescence-activated cell sorting analysis also showed that miR-365 overexpression blocked IGF-1-induced G1/S transition ( Supplementary Fig. S3i ). Furthermore, the upregulation of cyclin D1 and cdc25A upon IGF-1 stimulation was dramatically suppressed by miR-365 overexpression, and inhibition of miR-365 clearly restored the depressed expression of cyclin D1 and cdc25A upon LY294002 treatment ( Supplementary Fig. S3j,k ). Taken together, these results demonstrate that Akt signaling promotes GC cell proliferation at least partially through suppressing miR-365 expression. Akt suppresses miR-365 transcription by decreasing p53 We next asked which transcription factor downstream of the Akt pathway mediated the transcriptional regulation of miR-365. Previous studies have reported that miR-365 transcription is positively regulated by the transcription factors Sp1 and NF-κB to participate in host defense [34] or by the transcription factor Pparα to promote brown fat differentiation [33] . However, which transcription factor governs the ability of miR-365 to act as a tumour suppressor is unknown. We analysed the miR-193b-365 promoter [33] , [34] using rVista2.0 and found an evolutionarily conserved putative p53-binding site at the 801-bp upstream of the miR-193b-365 cluster. Previous studies have shown that activated Akt phosphorylates MDM2, which in turn stimulates p53 degradation [35] , [36] . Indeed, FBS or IGF-1 treatment repressed p53 abundance, whereas LY294002 induced higher p53 levels in BGC-823 cells ( Fig. 4a ), suggesting that Akt signaling downregulated p53 in GC cells. Furthermore, p53 was dramatically downregulated in PTEN -mutant epithelium ( Fig. 4b ). 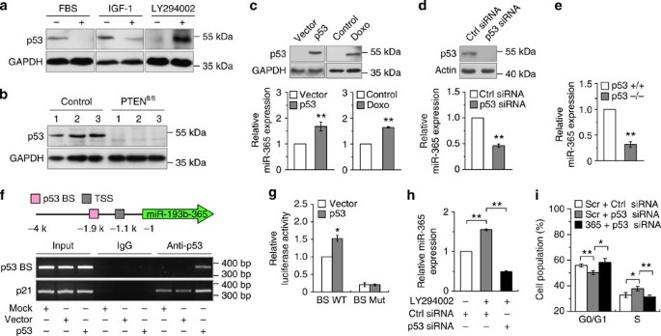Figure 4: Akt downregulates miR-365 in a p53-dependent manner. (a) The protein level of p53 was measured using western blot analysis in BGC-823 cells treated with FBS, IGF-1 or LY294002 (n=3). (b) The protein level of p53 was measured using western blot in thePTEN-mutant and control epithelium at P20 (n=5). (c,d) The relative level of miR-365 was measured using qRT–PCR in BGC-823 cells upon the change of p53 expression (n=4). p53 abundance was verified using western blot from the same cell lysates. (c) Cells were transfected with pCMV-Neo-Bam-p53 vector for 24 h or treated with doxorubicin (1 μM) for 12 h (n=6). (d) Cells were transfected with p53 or control siRNA for 48 h (n=3). (e) The relative level of miR-365 was measured using qRT–PCR inp53mutant and control epithelium at P20 (n=4). (f) ChIP assay detecting the binding of p53 to the miR-193b-365 promoter (n=3). BGC-823 cells were transfected with pCMV-Neo-Bam-p53 plasmid for 24 h. The p21 promoter was the positive control. A schematic diagram (upper) shows the promoter region of miR-193b-365 cluster in the genomic region and the luciferase vector containing the 4-kb region, in which the transcriptional start site (TSS) is represented as a black box and the p53-binding site (BS) as a pink box. (g) The luciferase reporter assay of the miR-193b-365 promoter constructs (n=5). BGC-823 cells were cotransfected with wild-type miR-193b-365 promoter construct (BS-WT) or p53-binding-site-mutant construct (BS-mut) with pCMV-Neo-Bam-p53. (h) The relative level of miR-365 was measured using qRT–PCR (n=4). BGC-823 cells were transfected with p53 siRNA for 36 h, followed by LY294002 addition for another 12 h. (i) Flow cytometry analysis detecting the distribution of the population to the different cell cycle stages (n=5). BGC-823 cells were cotransfected with miR-365 (365) or scrambled (Scr) mimic and p53 or control siRNA for 48 h. Values represent the mean±s.d. *P<0.05 and **P<0.01 were calculated using Student’st-test. Figure 4: Akt downregulates miR-365 in a p53-dependent manner. ( a ) The protein level of p53 was measured using western blot analysis in BGC-823 cells treated with FBS, IGF-1 or LY294002 ( n= 3). ( b ) The protein level of p53 was measured using western blot in the PTEN -mutant and control epithelium at P20 ( n= 5). ( c , d ) The relative level of miR-365 was measured using qRT–PCR in BGC-823 cells upon the change of p53 expression ( n= 4). p53 abundance was verified using western blot from the same cell lysates. ( c ) Cells were transfected with pCMV-Neo-Bam-p53 vector for 24 h or treated with doxorubicin (1 μM) for 12 h ( n= 6). ( d ) Cells were transfected with p53 or control siRNA for 48 h ( n= 3). ( e ) The relative level of miR-365 was measured using qRT–PCR in p53 mutant and control epithelium at P20 ( n= 4). ( f ) ChIP assay detecting the binding of p53 to the miR-193b-365 promoter ( n= 3). BGC-823 cells were transfected with pCMV-Neo-Bam-p53 plasmid for 24 h. The p21 promoter was the positive control. A schematic diagram (upper) shows the promoter region of miR-193b-365 cluster in the genomic region and the luciferase vector containing the 4-kb region, in which the transcriptional start site (TSS) is represented as a black box and the p53-binding site (BS) as a pink box. ( g ) The luciferase reporter assay of the miR-193b-365 promoter constructs ( n= 5). BGC-823 cells were cotransfected with wild-type miR-193b-365 promoter construct (BS-WT) or p53-binding-site-mutant construct (BS-mut) with pCMV-Neo-Bam-p53. ( h ) The relative level of miR-365 was measured using qRT–PCR ( n= 4). BGC-823 cells were transfected with p53 siRNA for 36 h, followed by LY294002 addition for another 12 h. ( i ) Flow cytometry analysis detecting the distribution of the population to the different cell cycle stages ( n= 5). BGC-823 cells were cotransfected with miR-365 (365) or scrambled (Scr) mimic and p53 or control siRNA for 48 h. Values represent the mean±s.d. * P <0.05 and ** P <0.01 were calculated using Student’s t -test. Full size image We further investigated whether p53 could regulate miR-365 transcription. In GC cell lines including BGC-823, AGS, NCI-N87 and PHM82, miR-365 expression was significantly upregulated by overexpression of wild-type p53 ( Fig. 4c ) or doxorubicin-induced p53 ( Fig. 4c ) but not by overexpression of mutant p53R175H ( Supplementary Fig. S4a,b ). Reciprocally, a significant reduction in miR-365 was observed in BGC-823 cells transfected with p53 siRNA ( Fig. 4d ). Additionally, miR-365 expression was greatly downregulated in the gastric epithelium of p53 knockout mice ( Fig. 4e ). Next, we examined whether p53 could physically interact with the putative p53-binding site of miR-365 promoter. Chromatin immunoprecipitation (ChIP) assays revealed that the specific PCR products derived from the p53-binding site were dramatically increased after p53 upregulation in BGC-823 ( Fig. 4f ) and HEK 293T cells ( Supplementary Fig. S4c,d ). Consistent with the ChIP assay result, luciferase reporter assays showed that p53 increased the luciferase activity of wild-type miR-193b-365 promoter by twofold but not the binding-site-mutant promoter ( Fig. 4g ). We further determined whether p53 mediated the negative regulation of Akt signaling on miR-365 expression. The luciferase reporter assays showed that the miR-193b-365 promoter carrying a mutant p53-binding site failed to reveal any response to activated or depressed Akt signaling ( Supplementary Fig. S4e ), indicating that the regulation of miR-365 expression by Akt signaling was largely dependent on p53. Furthermore, knockdown of p53 using siRNA rescued LY294002-induced upregulation of miR-365 expression ( Fig. 4h ). Moreover, overexpression of miR-365 blunted the effect of p53 knockdown on the cell cycle ( Fig. 4i ), and western blot results confirmed that knockdown of miR-365 partially rescued doxorubicin-induced downregulation of cyclin D1 and cdc25A ( Supplementary Fig. S4f,g ). In addition, etoposide-induced apoptosis was unchanged after miR-365 knockdown, indicating that p53-mediated apoptosis is miR-365-independent ( Supplementary Fig. S4h ). Collectively, our results suggest that p53 is required for Akt-regulated miR-365 transcription. Ablation of Akt1 inhibits PTEN -loss-driven tumour growth To investigate the involvement of the Akt-p53-miR-365 axis in gastric tumorigenesis driven by PTEN deficiency, we reduced the cellular pool of Akt protein and activity by breeding SP-A-Cre;PTEN fl/fl mice with Akt1 conditional knockout mice ( Akt1 fl/fl ) [37] . All SP-A-Cre;PTEN fl/fl ;Akt1 fl/fl compound-mutant mice displayed an improvement in survival, as evidenced by a lifespan >6 months ( Fig. 5a ). Histological examination revealed that 120-day-old SP-A-Cre;PTEN fl/fl ;Akt1 fl/fl double-mutant gastric epithelium exhibited dramatically reduced hyperplasia compared with that of the 50-day-old PTEN single knockout epithelium ( Fig. 5b ). BrdU-labelling results also showed that the proliferating cells in SP-A-Cre;PTEN fl/fl ;Akt1 fl/fl epithelium was significantly decreased compared with PTEN -mutant mice ( Fig. 5b ). As expected, simultaneous Akt1 deletion strikingly upregulated the abundance of p53 and miR-365 and downregulated the expression of cyclin D1 and cdc25A ( Fig. 5c,d ). These results indicated a possibility that concurrent deletion of Akt1 in PTEN -mutant mice leads to a markedly reduced cell proliferation because of, at least in part, the restored miR-365 expression. 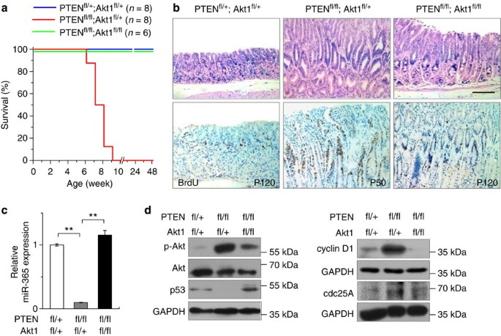Figure 5: Ablation of Akt1 suppressesPTEN-deletion-driven gastric tumour growth. (a) Survival curves ofSP-A-Cre;PTENfl/fl;Akt1fl/flmice (green;n=6),SP-A-Cre;PTENfl/+;Akt1fl/+control mice (blue;n=8) andSP-A-Cre;PTENfl/fl;Aktfl/+mice (red;n=8). (b) HE (upper) and BrdU-labelling assay (lower) of 120-day-oldSP-A-Cre;PTENfl/fl;Akt1fl/flandSP-A-Cre;PTENfl/+;Akt1fl/+along with 50-day-oldSP-A-Cre;PTENfl/fl;Akt1fl/+gastric epithelium. Scale bar represents 100 μm. (c) miR-365 expression in 120-day-oldAkt1andPTENdouble and control mice along with 50-day-oldPTENsingle mutant gastric epithelium determined using qRT–PCR (n=3).**P<0.01 calculated using Student’st-test. (d) Western blot analysis in gastric epithelium of 120-day-oldSP-A-Cre;PTENfl/+;Akt1fl/+controls andSP-A-Cre;PTENfl/fl;Akt1fl/fldouble homozygous mutants, as well as 50-day-oldSP-A-Cre;PTENfl/fl;Akt1fl/+mutants (n=4). Figure 5: Ablation of Akt1 suppresses PTEN -deletion-driven gastric tumour growth. ( a ) Survival curves of SP-A-Cre;PTEN fl/fl ;Akt1 fl/fl mice (green; n =6), SP-A-Cre;PTEN fl/+ ;Akt1 fl/+ control mice (blue; n =8) and SP-A-Cre;PTEN fl/fl ;Akt fl/+ mice (red; n =8). ( b ) HE (upper) and BrdU-labelling assay (lower) of 120-day-old SP-A-Cre;PTEN fl/fl ;Akt1 fl/fl and SP-A-Cre;PTEN fl/+ ;Akt1 fl/+ along with 50-day-old SP-A-Cre;PTEN fl/fl ;Akt1 fl/+ gastric epithelium. Scale bar represents 100 μm. ( c ) miR-365 expression in 120-day-old Akt1 and PTEN double and control mice along with 50-day-old PTEN single mutant gastric epithelium determined using qRT–PCR ( n= 3). ** P <0.01 calculated using Student’s t -test. ( d ) Western blot analysis in gastric epithelium of 120-day-old SP-A-Cre;PTEN fl/+ ;Akt1 fl/+ controls and SP-A-Cre;PTEN fl/fl ;Akt1 fl/fl double homozygous mutants, as well as 50-day-old SP-A-Cre;PTEN fl/fl ;Akt1 fl/+ mutants ( n =4). Full size image Orthotopic miR-365 represses gastric cell proliferation To determine whether miR-365 restoration could be truly beneficial for inhibiting gastric epithelial proliferation caused by PTEN deletion, we treated the PTEN- deficient mice with orthotopic injection of miR-365 mimic into the ventral submucosa and control scrambled mimic into the opposite dorsal submucosa ( Fig. 6a ). Although the levels of p-Akt of both sides were comparable after miR-365 injection ( Fig. 6c ), miR-365 levels increased by 7.6-fold in miR-365-mimic-injected epithelium compared with the opposite control mimic-injected region or by threefold compared with the control-mimic-treated wild-type epithelium ( Fig. 6b ). After four rounds of mimic treatment for 16 days ( Fig. 6a ), the miR-365-treated epithelium exhibited reduced hyperplasia compared with the control-mimic-treated one, as confirmed by a significant decrease in BrdU-labelling cells ( Fig. 6c ). As expected, miR-365 overexpression markedly decreased the expression of cyclin D1 and cdc25A ( Fig. 6c,d ) in gastric epithelium. These results indicated that miR-365 restoration decreases gastric cell proliferation induced by PTEN loss. 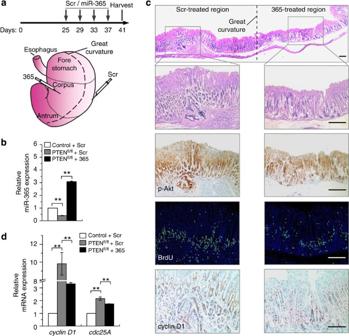Figure 6: Restoration of miR-365 repressesPTEN-deficient-induced hyperplasia. (a) Schematic of orthotopic miRNA injection protocols. Beginning at P25, 50 μg (5 μg μl−1) miR-365 mimic was injected into the ventral submucosa ofPTEN-mutant gastric corpus, and 50 μg control mimic was injected into the opposite dorsal submucosa, every 4 days for 16 days. (b)miR-365expression was detected using qRT–PCR 3 days after injection (n=3). (c) HE and immunohistochemical analysis of the expression of p-Akt, BrdU and cyclin D1 in miR-365 and control mimic-injected gastric epithelium (n=5). Scale bar represents 100 μm. (d) The expression ofcyclin D1andcdc25Awas detected using qRT–PCR in miR-365 and control mimic-injected gastric epithelium (n=5). Values represent the mean±s.d. *P<0.05 and **P<0.01 were calculated using Student’st-test. Figure 6: Restoration of miR-365 represses PTEN -deficient-induced hyperplasia. ( a ) Schematic of orthotopic miRNA injection protocols. Beginning at P25, 50 μg (5 μg μl −1 ) miR-365 mimic was injected into the ventral submucosa of PTEN -mutant gastric corpus, and 50 μg control mimic was injected into the opposite dorsal submucosa, every 4 days for 16 days. ( b ) miR-365 expression was detected using qRT–PCR 3 days after injection ( n =3). ( c ) HE and immunohistochemical analysis of the expression of p-Akt, BrdU and cyclin D1 in miR-365 and control mimic-injected gastric epithelium ( n =5). Scale bar represents 100 μm. ( d ) The expression of cyclin D1 and cdc25A was detected using qRT–PCR in miR-365 and control mimic-injected gastric epithelium ( n =5). Values represent the mean±s.d. * P <0.05 and ** P <0.01 were calculated using Student’s t -test. Full size image Reduced miR-365 expression in human GCs The above in vitro and in vivo evidence indicated that miR-365 acts as a suppressor in gastric tumorigenesis; we further tested whether altered miR-365 expression was possibly associated with human GCs. We examined miR-365 expression in 127 primary GC samples using qRT–PCR. A total of 76.4% (97/127) of patient tissues displayed lower miR-365 expression in tumour than adjacent normal tissues ( Fig. 7a ; Table 1 ). To further assess the correlations between miR-365 values and standard clinicopathological variables, the 127 clinical cases were divided into two groups: the low miR-365 group (T<N, n= 97) in which miR-365 expression was lower in tumour than in adjacent normal tissues and the high miR-365 group (T>N, n= 30) in which the miR-365 expression was higher in the tumour than in adjacent normal tissues. As shown in Table 1 , the decreased miR-365 expression significantly associated with poorly differentiated histology, deep invasion and advanced stage. To further define the clinical relevance of our finding that PTEN -deficiency-induced Akt activation repressed miR-365 expression by suppressing p53 abundance, we also detected the expression levels of miR-365’s upstream regulators PTEN, p-Akt and p53, as well as its downstream targets cyclin D1 and cdc25A in patient tissues using qRT–PCR or western blot. miR-365 expression was positively correlated with PTEN ( Fig. 7b ; Supplementary Fig. S5a ) and p53 levels ( Table 2 ) and negatively correlated with p-Akt levels ( Table 2 ). Moreover, an inverse correlation between miR-365 and cyclin D1 expression or cdc25A expressions was identified in patient samples ( Fig. 7c,d ; Supplementary Fig. S5b ). 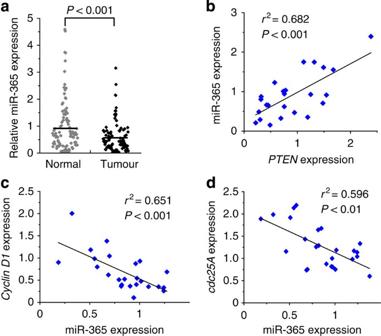Figure 7: Reduced miR-365 levels correlate with its upstream regulators and downstream targets in human gastric cancers. (a) The relative level ofmiR-365in 127 human gastric tumour tissues (black) and matched normal tissues distal to tumour regions (grey) detected using qRT–PCR. The band represents the mean.P<0.001 was calculated using Pair-Samplet-test. (b) A correlation between miR-365 and PTEN expression was determined using Spearman coefficient analysis in human gastric tumour tissues (n=24,r2=0.682,P<0.001). (c,d) Correlations between miR-365 and cyclin D1 or cdc25A expression were determined using Spearman coefficient in human gastric tumour tissues (cyclin D1:n=24,r2=0.651,P<0.001; cdc25A:n=25,r2=0.596,P<0.01). Figure 7: Reduced miR-365 levels correlate with its upstream regulators and downstream targets in human gastric cancers. ( a ) The relative level of miR-365 in 127 human gastric tumour tissues (black) and matched normal tissues distal to tumour regions (grey) detected using qRT–PCR. The band represents the mean. P <0.001 was calculated using Pair-Sample t -test. ( b ) A correlation between miR-365 and PTEN expression was determined using Spearman coefficient analysis in human gastric tumour tissues ( n =24, r 2 =0.682, P <0.001). ( c , d ) Correlations between miR-365 and cyclin D1 or cdc25A expression were determined using Spearman coefficient in human gastric tumour tissues (cyclin D1: n =24, r 2 =0.651, P <0.001; cdc25A: n =25, r 2 =0.596, P <0.01). Full size image Table 1 The correlations between miR-365 expression and clinicopathological characteristics of human gastric cancers. Full size table Table 2 Expression of p-Akt and p53 relative to miR-365 in human gastric cancers. Full size table The present study provides the first critical in vivo evidence showing a causal link between the activation of Akt signaling induced by PTEN deficiency and gastric tumorigenesis. We show that activated Akt signaling triggers gastric cell proliferation and tumorigenesis by downregulating miR-365 in a p53-dependent manner. Furthermore, we demonstrate that genetic deletion of Akt1 or local restoration of miR-365 expression significantly decreases gastric cell proliferation in PTEN -mutant mice, providing important implications for the treatment of PTEN -deficient GCs. We provide the first genetic evidence that PTEN deletion has a critical role in the initiation of gastric tumorigenesis. Using the SP-A-Cre transgenic mice, we restricted PTEN deletion to glandular epithelial cells rather than microenvironmental cells. We showed that loss of PTEN in gastric epithelial cells resulted in GC within the first 2 months of age, whereas concurrent ablation of Akt1 rescued the tumour growth induced by PTEN deficiency. Previous studies have revealed the dominant role of Akt1 in PTEN -deficiency-induced tumorigenesis including teratoma, endometrium neoplasia, prostate neoplasia, thyroid tumour, adrenal medulla tumour and intestinal polyps [38] , [39] . Our results demonstrated a cell-autonomous function of epithelial PTEN on suppressing gastric tumour formation and the role of intrinsic Akt overactivation in promoting gastric cell proliferation. Supportively, clinical observations show that in Cowden syndrome, 50% of patients carrying germline PTEN mutations have hyperplastic polyps in the gastrointestinal tract, including the stomach [40] , and in human GC samples, somatic PTEN deletion is often homogeneous [41] . These results strongly support the concept that loss of PTEN is an initiator in gastric tumorigenesis. The early onset and rapid progression of GC in PTEN -mutant mice indicated that PTEN -deleted gastric stem cells might contribute to gastric tumorigenesis. SP-A-Cre mice express Cre recombinase in whole gastric epithelium including putative stem cells from embryonic day 18.5. Previous studies have shown that CD44 and Lgr5 mark gastrointestinal stem cells that have significantly expanded in genetic mouse models for gastric or intestinal tumorigenesis [30] , [31] , [42] . Clinically, CD44 is a marker for GC stem cells [43] , and both CD44 and Lgr5 expression levels are correlated with human GC progression [44] , [45] , [46] , [47] . Of note, we found that PTEN deletion resulted in a significantly increased number of CD44- and Lgr5-positive cells, providing a possibility that PTEN could maintain gastric tissue homeostasis by suppressing the self-renewing activity of normal stem cells or the formation of GC stem cells. Supportively, previous studies have demonstrated the function of PTEN in the maintenance of the central nervous system and hematopoietic homeostasis by suppressing the self-renewing activity of neural stem cells [48] , [49] or restricting the activation of hematopoietic stem cells and inhibiting the formation of leukaemia stem cells [50] , [51] . Further dedicated studies are required to investigate the function of PTEN in the self-renewal and activation of gastric stem cells. We have verified the Akt-p53-miR-365-cyclin D1/cdc25A axis as a mechanism underlying gastric tumorigenesis caused by PTEN deficiency. Our results demonstrated that in GC cells, Akt activation suppresses p53 abundance, thereby leading to miR-365 downregulation and consequently resulting in the enhanced production of cyclin D1 and cdc25A. Furthermore, we provided a causal link between the Akt-p53-miR-365-cyclin D1/cdc25A axis and gastric carcinogenesis induced by PTEN loss in our mouse models. Genetic deletion of Akt1 or local restoration of miR-365 expression dramatically blocked PTEN -deficiency-induced hyperproliferation. In line with our findings, recent studies from colon and breast cancer cells have shown that Akt, through its downstream transcription factors C/EBP-β and p53, inhibits miR-145 expression [26] , [27] . These findings support the notion that Akt signaling could exert its oncogenic effect by downregulating a class of tumour-suppressive miRNAs. In the present study, we showed that in human GCs, aberrant expression of miR-365 was correlated with its upstream regulators PTEN, p-Akt, p53, as well as its targets cyclin D1 and cdc25A. These findings indicate that the PTEN-Akt-p53-miR-365-cyclin D1/cdc25A axis might be a therapeutic target for GC. A recent clinical phase I report shows that MK-2206, an oral inhibitor of all Akt isoforms, was effective in shrinking tumour volume in a patient with pancreatic adenocarcinoma [52] . In our study, Akt1 ablation efficiently reversed the hyperplasia in PTEN -mutant mouse, providing genetic evidence that Akt inhibitors may be a promising therapy for GC. Moreover, the efficiency of orthotopic miR-365 restoration by synthetic mimics in our mouse model underscored the potential application of miR-365 for GC therapy. Mice PTEN fl/fl mouse strain was provided by Dr Hong-Kui Deng, with kind permission from Dr Tak Wah Mak [28] . p53 −/− mouse was provide by Dr Chu-Xia Deng, with kind permission from Dr Lawrence A. Donehower [53] . ROSA26 transgenic mouse was provided by Dr Xiang Gao, with kind permission from Dr Philippe Soriano [54] . SP-A-Cre and Akt1 fl/fl mouse strains were previously generated [29] , [37] . Animal experiments were approved by the Animal Experiment Committee of the Institute of Biotechnology. Orthotopic injection of miRNA into mouse stomach Beginning at P25, mice received injection of miRNA mimic every 4 days, totally four rounds of injection. In details, Buprenorphine (Reckitt and Coleman Products, UK) was administered pre- and postoperatively at 0.09 mg kg −1 . Mice were anesthetized and their stomach was exposed. Under stereoscope, total 10 μl (5 μg μl −1 ) miR-365 mimic was injected into four spots of the corpus ventral submucosa and 10 μl (5 μg μl −1 ) control scrambled mimic into the opposite dorsal submucosa, through an insulin syringe with 31-gauge needle (BD Biosciences). Mice had excellent mobility within 2 h after the surgery. Human gastric tissues Paired advanced GC and adjacent non-tumour gastric tissues were obtained after review and approval by the Cancer Tissue Bank of the Affiliated Cancer Hospital of Zhengzhou University. Informed consent was obtained from each patient before operation. All sample data including age, gender, invasion depth, clinical stage and histological grade were obtained from the clinical and pathologic records. Histopathology and Immunostaining For LacZ staining, stomach tissues were fixed in 4% paraformaldehyde for 2 h and subjected to LacZ staining. Immunohistochemistry analysis was carried out on paraffin-embedded sections, and Immunofluorescent analysis was carried out on cryostat sections. The primary antibodies and lectin used in this study were as follows: pepsinogen II (1:100; Abcam; ab9013), bromodeoxyuridine (BrdU; 1:300; Abcam; ab6326), PTEN (1:100; CST; no. 9188), p-Akt (1:100; CST; no. 4060), cyclin D1 (1:100; Epitomics; 2261), CD44 (1:40; BD Biosciences; 550538), TRITC-labelled UEA (1:100; Sigma; L4889), FITC-labelled DBA (1:100; Sigma; L9142) and biotinylated GS II (1:100; Vector Laboratories; B-1215). For BrdU labelling, mice were intraperitoneally injected with 100 mg g −1 body weight of BrdU 2 h before killing. In situ hybridization In situ hybridization was performed on paraffin sections The lgr5 probe was amplified by sense primer 5′-CTGGAGCAAAGATCTCATCTC-3′ and antisense primer 5′-GGGACGATCACGAGAAGTATA-3′, and labelled with 35 S-UTP. Slides were dipped in photographic emulsion (Amersham Pharmacia) and exposed for 3–10 days. Microarray experiments The miRNA expression profiling was measured using microarray analysis performed by LC Sciences (Houston, TX) ( http://lcsciences.com/ ). Differentially detected signals were those with <0.01 P -value. ( GSE27047 ) record can be found at http://www.ncbi.nlm.nih.gov/geo/query/acc.cgi?acc=GSE27047 . Cell culture and treatment The cell lines HEK 293T and AGS were obtained from the American Type Culture Collection (ATCC). BGC-823 cell line was from Dr. Ying-Ge Zhang. SGC-790, PHM82 and NCI-N87 cell lines were from Dr. Ming-Zhou Guo. The above cell lines were cultured in Dulbecco's Modified Eagle Medium or Roswell Park Memorial Institute formulation 1640 supplemented with 10% FBS (Hyclone). For nocodazole treatment, cells were incubated with nocodazole (100 ng ml −1 ; Sigma-Aldrich) for 20 h. Establishment of transiently and stably transfected cells Cells were individually plated on tissue culture plates or dishes 24 h before transfection. Transient transfection of miRNA mimic or antisense oligonucleotides (anti-) and control oligonucleotides of scrambled sequence (Scr) (Genepharm) at a final concentration of 50 nM was accomplished with lipofectmine2000 reagent (Invitrogen). The cyclin D1 expression vector was constructed by inserting human cyclin D1 cDNA into the pCMV-HA vector (pCMV-HA-cyclin D1). The pCMV-HA-cyclin D1, pCMV6-cdc25A-GFP (ORIGENE; 200496), pCMV-Neo-Bam-p53 (Addgene) andpUSE-myr-Akt1 (Millipore) transfections were used at a final concentration of 2 μg ml −1 . The Akt siRNA (CST; no. 6211), p53 siRNA (CST; no. 6512), cyclin D1 siRNA (Santa Cruz; SC-29286) and cdc25A siRNA (Santa Cruz; SC-29254) were transfected with a final concentration of 100 nM. To establish stably transfected AGS and BGC-823 cell lines, the 626-bp genomic sequence of miR-365 precursor was inserted into the pIRES2-EGFP vector (Clontech). The PCR primers for miR-365 precursor are as follows: sense, 5′-CCGCTCGAGAGGGTCTGGAACAGTCATC-3′, antisense, 5′-CCGGAATTCAAAGCACGTTTAGCAACC-3′. Stably transfected cells were selected using G418 (500 μg ml −1 , Gibco). Proliferation and colony formation assays For the proliferation assay, 2 × 10 4 cells were seeded onto 24-well plate in triplicate, and cell number was counted under microscope using a hemocytometer at different time points. For the plate colony formation assay, 5 × 10 2 stably or transiently transfected cells independently were plated onto six-well plates. After 10 days, visible colonies were fixed with methanol and stained with Crystal violet. For soft agar colony formation assays, 2 × 10 3 stably miR-365-expressing BGC-823 cells or control cells were seeded and grown in soft agar for 20 days. Colony with diameter >100 μm was counted using microscopic inspection. Tumorigenicity in nude mice Stably miR-365-expressing BGC-823 and control cells (1.0 × 10 6 ) were suspended in 100 μl phosphate-buffered saline and then injected subcutaneously into either side of the back of the same female BALB/c nude mouse at the age of 4–5 weeks. Tumour growth was examined about 4 weeks later. Tumour volume ( V ) was monitored by measuring the length ( L ) and width ( W ) with calipers and calculated with the formula ( L × W 2 )/2. Luciferase activity assay The 3′-UTR regions of human cyclin D1 and cdc25A that contain the miR-365-binding sites were amplified using the following specific primers: cyclin D1 sense, 5′-CCGCTCGAGATACCAGAAGGGAAAGCT-3′; cyclin D1 antisense, 5′-CCGACGCGTCAGGCTGAATCAATGTCT-3′; cdc25A sense, 5′-CCGCTCGAGTGCCTGACATAAGCTAAAT-3′; cdc25A antisense, 5′-CCGACGCGTAACTCAAACCCGTAACAC-3′. Overlapping PCR was performed to mutate six bases of seed sequence in miR-365-binding sites, using additional two pair of primers: cyclin D1 mut sense, 5′-CCGCCATGGAACACAAAGGAGGCGTCTCG-3′; cyclin D1 mut antisense, 5′-CCGCCATGGTATTCTTACAACAGAGAAACAAG-3′; cdc25A mut sense, 5′-CCGGAATTCAGGAGAAGGGAGTGGGTGC-3′; cdc25A mut antisense, 5′-CCGGAATTCCAGGGCTTCCAGCCCCTC-3′. Luciferase activity assays were performed at 48 h after transfection using a Dural-luciferase reporter assay system (Promega) using LB 960 Centro XS3 luminometer (Berthold Technologies). Quantitative Real-time PCR The miRNA qRT–PCR was performed using the TaqMan miRNA Reverse Transcription Kit (Applied Biosystems) and the LightCycler Real-Time PCR System (Roche). The data were normalized by comparing with U6. The mRNA qRT–PCR was performed using the LightCycler Real-Time PCR System (Roche). Primers: PTEN-human-sense: 5′-TGGATTCGACTTAGACTTGACCT-3′; PTEN-human-antisense: 5′-TGGCGGTGTCATAATGTCTTTC-3′; cyclin D1-human-sense, 5′-GCTGCGAAGTGGAAACCATC-3′; cyclin D1-human-antisense, 5′-CCTCCTTCTGCACACATTTGAA-3′; cdc25A-human-sense, 5′-GTGAAGGCGCTATTTGGCG-3′; cdc25A-human-antisense, 5′-GGTCCATAGTGACGGTCAGGT-3′; cyclin D1-mouse-sense, 5′-GCGTACCCTGACACCAATCTC-3′; cyclin D1-mouse-antisense, 5′-ACTTGAAGTAAGATACGGAGGGC-3′; cdc25A-mouse-sense, 5′-TCCCTGACGAGAATAAATTCCCT-3′; cdc25A-mouse-antisense, 5′-TCGATGAGGTGAAAGGTGTCG-3′. Immunoblotting Immunoblotting was performed using the following antibodies: PTEN (1:1,000; CST; no. 9188), Akt (1:1,000; CST; no. 4685), p-Akt (1:1,000; CST; no. 4060), cdc25A (1:1,000; CST; no. 3652), cdc25A (1:1,000; Santa Cruz; 7389), p53 (1:1,000; Santa Cruz; 71818), p53 (1:1,000; CST; no. 2524, no. 2527), cyclin D1 (1:1,000; Epitomics; 2261), GAPDH (1:1,000; ZSGB-Bio; TA-08) and β-actin (1:1,000; Sigma; SC-1615). ChIP assay ChIP was performed using a ChIP kit (Upstate Biotechnology). DNA–protein complexes were immunoprecipitated using anti-p53 antibody (CST; no. 2527). The specific primers for p53-binding site of miR-193b-365 cluster promoter are as follows: sense, 5′-GCGAGCGTTTCTAGGAAGGC-3′, antisense, 5′-CCCAGACGAGATCCAAGTGATG-3′. Statistical analysis All values were expressed as mean±s.d. Statistical analysis was performed using two-tailed Student’s t- test or χ 2 test, and results were considered statistically significant at P <0.05. Statistical significance of correlation was calculated using Spearman correlation analysis. Accession codes: The microarray data have been deposited in the Gene Expression omnibus under accession code GSE27047. How to cite this article: Guo, S.-L. et al . Akt-p53-miR-365-cyclin D1/cdc25A axis contributes to gastric tumorigenesis induced by PTEN deficiency. Nat. Commun. 4:2544 doi: 10.1038/ncomms3544 (2013).